Assembly of complex plant–fungus networks Species in ecological communities build complex webs of interaction. Although revealing the architecture of these networks is fundamental to understanding ecological and evolutionary dynamics in nature, it has been difficult to characterize the structure of most species-rich ecological systems. By overcoming this limitation through next-generation sequencing technology, we herein uncover the network architecture of below-ground plant–fungus symbioses, which are ubiquitous to terrestrial ecosystems. The examined symbiotic network of a temperate forest in Japan includes 33 plant species and 387 functionally and phylogenetically diverse fungal taxa, and the overall network architecture differs fundamentally from that of other ecological networks. In contrast to results for other ecological networks and theoretical predictions for symbiotic networks, the plant–fungus network shows moderate or relatively low levels of interaction specialization and modularity and an unusual pattern of ‘nested’ network architecture. These results suggest that species-rich ecological networks are more architecturally diverse than previously recognized. Interactions among species form networks that, although complex, show repeatable patterns in species-rich communities [1] , [2] , [3] . Although the overall ecological and evolutionary dynamics of these networks follow from some basic predictions of network theory [3] , [4] , [5] , the distribution and organization of links (that is, interactions) among species and their community-scale consequences often vary among different forms of interaction [3] , [6] . How and why the architecture of these networks varies in nature has therefore become an increasingly important problem, especially at a time when the species composition of communities worldwide is changing at unprecedented rates. Ecological networks are usually compartmentalized into modules of closely interacting species, and the modules are in turn connected by a few supergeneralist (that is, hub) or connector species [2] , [5] . A potential key factor that determines the number, size and distribution of modules within ecological networks is the intimacy of interspecific interactions [7] , [8] , [9] . Most studies of network structure have targeted interactions among free-living species such as plants and their pollinators or seed dispersers or predators and prey [2] , [3] , [10] . In contrast to these interactions, those between hosts and their parasites, parasitoids, commensalists or mutualistic symbionts involve intimate and long-lasting relationships: hereafter, we use the word ‘symbionts’ in the broad sense [9] to refer to all those antagonistic, commensalistic and mutualistic organisms on/within hosts. Coevolution acting on these intimate interactions is predicted to lead to greater reciprocal specialization among partners than coevolution among free-living species, resulting in networks that differ in structure and patterns of ongoing evolutionary change [9] , [11] . Some empirical studies have shown that species with symbiotic interactions are, in fact, more specialized and modular than those with non-symbiotic (free-living) interactions [7] , [8] , but these results mostly come from networks involving limited taxonomic groups of interacting species. The lack of knowledge of large symbiotic networks has therefore hindered us from understanding the full span of determinants of ecological network architecture. Recent technical breakthroughs, however, are enabling the investigation of species-rich ecological networks involving functionally and phylogenetically diverse symbiont/parasite taxa, thereby providing new opportunities for characterizing network structure more accurately and precisely. Here we analyse a massive next-generation sequencing data set [12] of plant–fungus associations in a temperate forest in Japan, by testing whether networks of plants and their functionally and phylogenetically diverse root-associated fungi have architectural properties consistent with or different from those of other symbiotic and non-symbiotic networks. These below-ground plant–fungus symbioses are among the most ubiquitous symbiotic interactions found in terrestrial ecosystems [12] , [13] , [14] , [15] . More than 90% of all plant species interact with diverse groups of mycorrhizal fungi (for example, ectomycorrhizal and arbuscular mycorrhizal fungi), which enhance plant survival and growth rate [13] . In addition to mycorrhizal fungi, plant roots are ubiquitously colonized by diverse endophytic fungi [16] , some of which are known to increase host plant fitness [17] . Thus, a plant community, besides being involved in well-studied pollination and seed dispersal networks [1] , [10] , is also involved in another important mutualistic network with functionally and phylogenetically diverse fungi. Our analysis indicates that the large plant–fungus network has architectural properties fundamentally different from those of previously investigated ecological networks. In particular, despite the fact that most previously investigated plant–mutualistic partner networks have nested interaction architecture [1] , [3] , the nestedness of the plant–fungus network is lower than expected under null models of random associations. This result is further supported by additional statistical tests in which we consider potential effects of sampling intensity and criteria in next-generation sequencing analyses on the estimation of network architecture. As present ecological theories rely greatly on findings of network architectural structures in ecological interactions [3] , [4] , [6] , technological advances in analysis of ecological networks will continue to be needed to develop a more comprehensive understanding of ecological and coevolutionary processes at the level of network. Diversity within the network and connectance The network of symbiotic interactions between plant and fungal taxa ( Fig. 1 ; Supplementary Fig. 1 ) was highly asymmetric in species richness. It included fewer plant species than fungal operational taxonomic units (OTUs): 33 vs 387 (ref. 12 ), resulting in a mean of 27.7 fungal OTUs interacting per plant species. Although <8% of possible interactions actually occur (connectance=0.072), this proportion of the observed interactions among plant and fungal taxa was as high as or even slightly higher than those of previously reported large ecological networks ( Fig. 2a ). 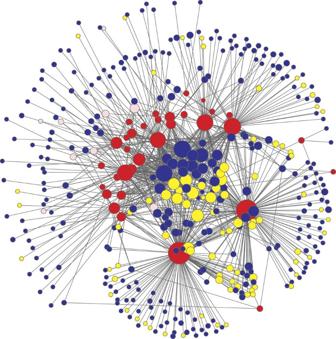Figure 1: Architecture of the below-ground plant–fungus network in a temperate forest in Japan. In the bipartite network, plant species (red) interact with ectomycorrhizal (yellow) and arbuscular mycorrhizal (pink) fungal OTUs as well as OTUs with unknown ecological functions (blue). The size of nodes represents the relative abundance of plant species or fungal OTUs in the data set12. Figure 1: Architecture of the below-ground plant–fungus network in a temperate forest in Japan. In the bipartite network, plant species (red) interact with ectomycorrhizal (yellow) and arbuscular mycorrhizal (pink) fungal OTUs as well as OTUs with unknown ecological functions (blue). The size of nodes represents the relative abundance of plant species or fungal OTUs in the data set [12] . 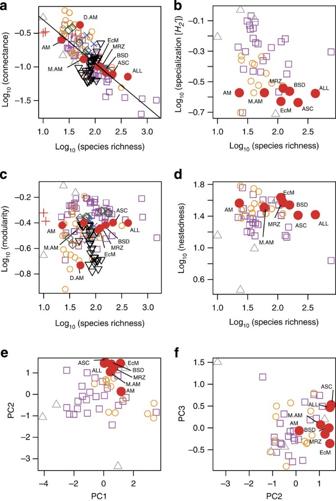Figure 2: Comparison of network architecture with other forms of ecological networks. (a) Network connectance. The symbols represent plant–pollinator (square, purple), plant–seed disperser (open circle, orange), myrmecophyte plant–ant (triangle, grey), anemone–anemonefish (plus, red), host–parasite (diamond, green), plant–herbivore (cross, blue), food web (reverse triangle, black) and plant–fungus (filled circle, red) networks. The regression line of the relationship between network size (species richness) and connectance is shown (log10(connectance), −0.644 × log10(species richness)+0.337;F1, 127, 180,P<0.0001 (ANOVA)). ALL, the entire network involving all plant species and fungal OTUs; AM, arbuscular mycorrhizal partial network; ASC, ascomycete partial network; BSD, basidiomycete partial network; D.AM, an arbuscular mycorrhizal network in Estonia14; EcM, ectomycorrhizal partial network; M.AM, an arbuscular mycorrhizal network in Mexico15and MRZ, mycorrhizal partial network. (b)H2′ network level specialization11of the 47 data sets with quantitative information of interaction frequency (c) network modularity and (d) nestedness (weighted NODF) for the 47 data sets with interaction frequency information. (e,f) Principal component analysis. Larger values in the principal component (PC) axis 1 represent highly nested (factor loading (r) for modularity=0.55) and connected (r=0.37) networks, whereas small values represent highly compartmentalized (r=−0.57) and specialized (r=−0.49) networks. High values in the PC axis 2 indicate low connectance (r=−0.82) and low specialization (r=−0.55) and the PC axis 3 is negatively correlated with nestedness (r=−0.81). Full size image Figure 2: Comparison of network architecture with other forms of ecological networks. ( a ) Network connectance. The symbols represent plant–pollinator (square, purple), plant–seed disperser (open circle, orange), myrmecophyte plant–ant (triangle, grey), anemone–anemonefish (plus, red), host–parasite (diamond, green), plant–herbivore (cross, blue), food web (reverse triangle, black) and plant–fungus (filled circle, red) networks. The regression line of the relationship between network size (species richness) and connectance is shown (log 10 (connectance), −0.644 × log 10 (species richness)+0.337; F 1, 127 , 180, P <0.0001 (ANOVA)). ALL, the entire network involving all plant species and fungal OTUs; AM, arbuscular mycorrhizal partial network; ASC, ascomycete partial network; BSD, basidiomycete partial network; D.AM, an arbuscular mycorrhizal network in Estonia [14] ; EcM, ectomycorrhizal partial network; M.AM, an arbuscular mycorrhizal network in Mexico [15] and MRZ, mycorrhizal partial network. ( b ) H 2 ′ network level specialization [11] of the 47 data sets with quantitative information of interaction frequency ( c ) network modularity and ( d ) nestedness (weighted NODF) for the 47 data sets with interaction frequency information. ( e , f ) Principal component analysis. Larger values in the principal component (PC) axis 1 represent highly nested (factor loading ( r ) for modularity=0.55) and connected ( r =0.37) networks, whereas small values represent highly compartmentalized ( r =−0.57) and specialized ( r =−0.49) networks. High values in the PC axis 2 indicate low connectance ( r =−0.82) and low specialization ( r =−0.55) and the PC axis 3 is negatively correlated with nestedness ( r =−0.81). Full size image Network architecture Plants and fungi in the network were associated with fewer other species than expected by chance. Specifically, the organization of the links in the plant–fungus network showed more specialization and unevenness than expected under the null models that assume that frequencies of interactions are the result of random associations of plants and fungi ( Fig. 3a ; Supplementary Fig. 2 ; Supplementary Table 1 ). In contrast to the general prediction that species in symbiotic systems should be more specialized than those in non-symbiotic systems [7] , [9] , the extent of interaction specialization was relatively low. The H 2 ′ estimate of interaction specialization [11] was 0.265, which was as low as those previously reported in plant–seed disperser networks (0.354±0.085, N =12) but much lower than those reported in plant–pollinator networks (0.533±0.170, N =24) ( Fig. 2b ; Supplementary Table 2 ). 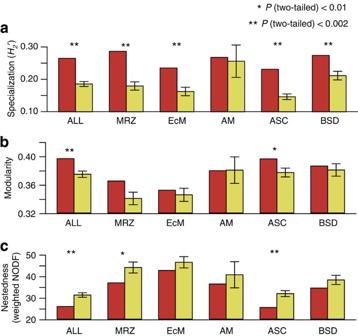Figure 3: Architectural properties of the plant–fungus network. (a)H2′ metric of network-level specialization. The observedH2′ metric of interaction specialization (left red bars) is shown for each network or partial network. Asterisks indicate significant deviation of observedH2′ values from those of randomized networks (right yellow bars (mean±s.d.)). (b) Modularity. (c) Nestedness (weighted NODF ). ALL, the entire network involving all plant species and fungal OTUs; AM, arbuscular mycorrhizal partial network; ASC=ascomycete partial network; BSD, basidiomycete partial network; EcM=ectomycorrhizal partial network; MRZ, mycorrhizal partial network. Figure 3: Architectural properties of the plant–fungus network. ( a ) H 2 ′ metric of network-level specialization. The observed H 2 ′ metric of interaction specialization (left red bars) is shown for each network or partial network. Asterisks indicate significant deviation of observed H 2 ′ values from those of randomized networks (right yellow bars (mean±s.d.)). ( b ) Modularity. ( c ) Nestedness (weighted NODF ). ALL, the entire network involving all plant species and fungal OTUs; AM, arbuscular mycorrhizal partial network; ASC=ascomycete partial network; BSD, basidiomycete partial network; EcM=ectomycorrhizal partial network; MRZ, mycorrhizal partial network. Full size image The plant–fungus network was more compartmentalized than expected by chance ( Fig. 3b ; Supplementary Table 1 ). We detected eight interconnected modules, which differed in their composition of fungal functional groups ( G -test; G =32.4, df=14, P =0.0035) and phylogenetic groups ( G =46.5, df=21, P =0.0011; Supplementary Fig. 3 ). For example, the module including the two oak species Quercus serrata and Q. glauca (module 3) had a high percentage of ectomycorrhizal fungal OTUs (29.7%), but no arbuscular mycorrhizal fungal OTUs ( Supplementary Fig. 3 ). A high proportion (41.3%) of the fungal OTUs in this module was Basidiomycota, as expected by the prevalence of ectomycorrhizal fungi in the fungal phylum. In contrast, the module encompassing Ilex , Prunus and Cinnamomum species (module 4) had a low percentage of ectomycorrhizal fungi (5.6%), but instead included several arbuscular mycorrhizal fungal taxa (7.0%). Ascomycota fungi dominated this module (64.8%; Supplementary Fig. 3 ). The network modularity ( M =0.397) was as high as that previously reported in host–parasite (symbiotic) networks (0.408±0.082, N =7), higher than that generally observed in plant–seed disperser networks (0.323±0.116, N =25) and food webs (0.274±0.075, N =27), but lower than that usually observed in plant–pollinator networks (0.451±0.108, N =51) ( Fig. 2c ). The plant–fungus network lacked an important and common architectural property, namely, nestedness [1] ( Fig. 3c ). Nestedness is commonly observed in ecological networks and considered an important property promoting species coexistence in mutualistic systems [3] , [4] , [18] . Within the overall plant–fungus network, interactions were not grouped as nested subsets, unlike in other mutualistic networks [1] ( Fig. 3c ). On the contrary, the nestedness of the plant–fungus network was even lower than expected by chance ( Fig. 3c ; Supplementary Table 1 ), as previously observed in some symbiotic associations involving fewer species [7] . Comparative analysis of network architecture We then conducted a detailed comparison of network architecture between the plant–fungus network and other symbiotic and non-symbiotic ecological networks. The H 2 ′ measure of interaction specialization differed among different forms of interactions (Kruskal–Wallis test; χ 2 =19.0, df=3, P =0.0003); the plant–fungus network and ‘partial’ networks (see below), including a plant–arbuscular mycorrhizal fungus network of a previous study [15] , were less specialized than plant–pollinator networks (Steel-Dwass test; t =3.5, P =0.002; Fig. 2b ). Although modularity and nestedness estimates varied significantly among different forms of interactions (modularity, χ 2 =45.7, df=7, P <0.0001; weighted NODF nestedness, χ 2 =12.1, df=3, P =0.007), those of plant–fungus networks/partial networks did not significantly differ from those of other symbiotic and non-symbiotic networks ( P >0.05; Fig. 2c,d ). The architectural features of the plant–fungus network were further compared with other symbiotic and non-symbiotic networks based on a principal component analysis ( Fig. 2e,f ; Supplementary Fig. 4 ; Supplementary Tables 3 and 4 ). Along the first principal component axis, plant–pollinator interactions displayed more compartmentalized and specialized network architecture than others, while plant–seed disperser interactions had a highly connected and nested network structure ( Fig. 2e,f ). The plant–fungus network/partial networks displayed intermediate properties in this respect. The second principal component axis represented a counterintuitive and unexplored combination of low connectance and low interaction specialization ( Supplementary Table 3 ), and the plant–fungus network/partial networks showed highest values along the axis ( Fig. 2e,f ). The third principal component axis was negatively correlated with nestedness ( Supplementary Table 3 ), and the plant–fungus network/partial networks displayed values as high as those of host–parasite networks ( Fig. 2e,f ). Functional and phylogenetic partial networks We next explored whether the remarkable diversity of fungi was responsible for the differences we found in this network in comparison with other networks of interacting species. Most studies of ecological networks have focused on a few functional or taxonomic groups such as the suite of insects visiting flowers [1] , [2] . The plant–fungus network, however, included functionally and phylogenetically diverse fungal taxa, whose interactions with host plants have been analysed separately in most previous mycological studies [13] . We compared our results with previous studies by examining the structure of each functional or phylogenetic ‘partial network’ ( Fig. 3 ; Supplementary Fig. 2 ; Supplementary Table 1 ). The observed architectural properties of the partial networks were largely consistent with those observed in the entire plant–fungus network ( Figs 2 and 3 ; Supplementary Figs 2 and 4 ; Supplementary Table 1 ). Inclusion of a previously studied arbuscular mycorrhizal network [15] in Mexico further underlined the architectural uniqueness of below-ground plant–fungus associations ( Fig. 2 ). Specifically, the links in the mycorrhizal and ascomycete partial networks were more specialized, and more uneven, and less nested than expected under the null model of random associations. This result is partially consistent with a recent report that interactions between plants and mycorrhizal fungi could display significantly low nestedness [19] , but careful interpretation is required when comparing these studies because the previous study on ectomycorrhizal symbioses analysed networks of only two to four plant species [19] . Modularity was again lower than that usually observed in plant–pollinator networks for the four of the partial networks examined and was significantly higher than expected by chance only for the ascomycete partial network. Previous studies have usually found significant modularity in ecological mutualistic networks with many species (283.9±249.0, N =29), but rarely in networks with few species (67.1±37.0, N =22) [2] , [20] . No network property was significant for the arbuscular partial network, presumably due to the small size of the partial network (13 plant species and 10 fungal OTUs). Cutoff DNA sequence similarities and network architecture We also examined the potential dependency of the result on the cutoff DNA sequence similarities defining fungal OTUs and obtained consistent results with different similarity threshold values ( Fig. 4 ; Supplementary Figs 5 and 6 ). This analysis allowed an assessment of how the degree of genetic difference among nodes affected the interpretation of network architecture. Varying the cutoff did not alter qualitatively the results, reinforcing the conclusion that these networks are organized in unique ways. 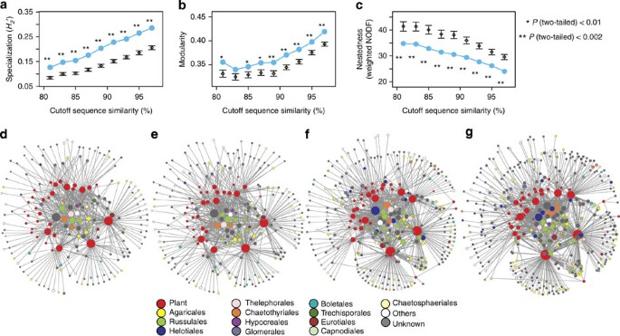Figure 4: Network architecture and cutoff sequence similarities defining fungal OTUs. With varying cutoff internal-transcribed-spacer (ITS) sequence similarities defining fungal OTUs (nodes), the randomization analysis of interaction specialization (a), modularity (b) and nestedness (c) was re-conducted. Asterisks indicate significant deviation of observed estimates (filled circles) from those of randomized networks (diamonds; mean±s.d.). The network topologies at 83% (d), 87% (e), 91% (f) and 95% (g) cutoff sequence similarities are also shown. The order level taxonomy of each fungal node is indicated by colour. Figure 4: Network architecture and cutoff sequence similarities defining fungal OTUs. With varying cutoff internal-transcribed-spacer (ITS) sequence similarities defining fungal OTUs (nodes), the randomization analysis of interaction specialization ( a ), modularity ( b ) and nestedness ( c ) was re-conducted. Asterisks indicate significant deviation of observed estimates (filled circles) from those of randomized networks (diamonds; mean±s.d.). The network topologies at 83% ( d ), 87% ( e ), 91% ( f ) and 95% ( g ) cutoff sequence similarities are also shown. The order level taxonomy of each fungal node is indicated by colour. Full size image Rarefaction analysis Although our data are based on 834 root samples, they were collected from a relatively small (59 m × 15 m) area in a forest [12] , and we therefore evaluated the degree to which our sampling captured local diversity. Rarefaction analysis of the data by 60% ( Supplementary Fig. 7 ) indicated stable estimates of H 2 ′, modularity and nestedness. The rarefaction analysis also indicated that about 500 root samples (~60% in our data set) were sufficient for characterizing the architectural properties (for example, significantly low nestedness) of these plant–root-associated fungus networks ( Supplementary Table 5 ). The characteristic network structure of below-ground plant–fungus networks ( Figs 2e,f and 3 ) may result from the unique biological features of these interactions. Unlike other symbiotic systems, a fungal symbiont individual can simultaneously interact with multiple host individuals in mycorrhizal interactions [21] , [22] . As reward levels provided by a host plant individual (for example, carbohydrates) change with the host’s physiological status or the soil nutrients available to the plants [13] , [21] , many mycorrhizal fungi are thought to have evolved wide rather than narrow ranges of host plants [23] . If fungi are phenotypically plastic and can abandon interactions with less profitable hosts depending on local biotic/abiotic environmental conditions [21] , [24] , natural selection would favour the ability to interact with a potentially broad range of hosts. The ability to use multiple plant species and the unique ability of fungi to interact simultaneously [9] , [13] may be partly responsible for the observed moderate modularity in below-ground plant–fungus symbiosis. Although many of the links in the network likely represent mutualistic interactions, especially those involving mycorrhizal fungi, the plant–fungus network may also include commensalistic and even antagonistic interactions. Diverse clades of root-endophytic and plant-pathogenic fungi are possibly present within the root-associated fungal community of the studied forest [12] , [16] . Non-mutualistic effects of partners are likely to occur even in interactions involving mycorrhizal fungi, as the benefit and cost of interacting with specific mycorrhizal hosts/symbionts depend on internal physiological status and/or abiotic/biotic environmental conditions [21] . Non-mutualistic links are likely part of all mutualistic networks. For example, the presence of cheaters (for example, nectar robbers) and the context-dependency of interaction type [25] are also expected in previously studied plant–pollinator interactions. Inclusion of these antagonistic links in the description of predominantly mutualistic ecological networks is meaningful, as the lifestyles of these antagonists rely on the existence of mutualistic networks and may affect the stability [26] and coevolutionary processes [9] of mutualisms. Thus, development of a comprehensive conceptual framework for understanding ecological and coevolutionary dynamics will require analysis of all types of possible interactions in a community [26] , [27] . While arbuscular mycorrhizal, ectomycorrhizal, endophytic and parasitic fungi are sampled and analysed separately in most mycological studies [13] , the present study indicates that compartmentalization by fungal functional or phylogenetic groups is incomplete in real ecological communities. This proposition is supported by recent studies showing that plant species can be simultaneously infected by both arbuscular and ectomycorrhizal fungi [28] and that fungal taxonomic clades can involve both mycorrhizal and endophytic species [29] . Of course, the present data set can include many links of weak, commensalistic or neutral interactions, and hence further technical advances that allow high-throughput evaluation of interaction type/strength are necessary. Ever since Darwin’s deliberation of an ‘entangled bank’ full of interacting species [30] , ecologists and evolutionary biologists have investigated how interspecific interactions are organized in biological communities. Although we have already had data sets of large predator–prey, plant–pollinator, and plant–seed disperser networks encompassing hundreds of species, those visible interactions represent only a tiny fraction of diverse interspecific interactions found in nature. By expanding the target of ecological network analysis to hyperspecies-rich symbiotic interactions by means of high-throughput sequencing, we have shown that the diversity of ecological network architecture has been underappreciated. The significantly low nestedness observed in the plant–fungus network is particularly important, as theoretical studies have argued that the commonly reported nested patterns in species networks could determine feasibility, resilience, persistence and structural stability of ecological communities [4] , [6] , [18] , [31] , [32] . A comprehensive understanding of the laws that organize the earth’s biosphere will require continued exploration of ecological network architecture in diverse symbiotic and non-symbiotic networks. Data As shown in an intensive study of Lepidopteran hosts and their parasitoids [33] , DNA-barcoding-based research of interspecific interactions not only enables the high-throughput and standardized data collection of interactions that have been recognized by traditional observational methods, but also allows us to find a number of novel ecological interactions, which had been difficult to detect with conventional methods [34] , [35] , [36] . By further expanding those DNA-barcoding analyses by means of next-generation sequencing, an analysis of root-associated fungi was conducted to understand how plants and their functionally and phylogenetically diverse fungal symbionts were associated with each other in a forest [12] . In principle, DNA-barcoding-based data sets of plant–root-associated fungus associations can include not only network links with mutually beneficial host–symbiont interactions but also links with potentially commensalistic or antagonistic interactions [12] , [37] . Thus, network theoretical analyses based on DNA-barcoding information require careful attention to the fact that host–symbiont links in a network data set could vary in their ecological effects [26] . This situation is possibly common to other ecological network studies: for example, the presence of non-efficient pollinators and/or nectar robbers is usual in the observational data sets of flower visitors [38] , [39] . The temperate secondary forest studied was located on Mt. Yoshida, Kyoto, Japan (35°02′N, 135°47′E), wherein evergreen and deciduous oak trees, Quercus glauca and Q. serrata (Fagaceae), are dominant and co-occur with evergreen trees such as Ilex pedunculosa (Aquifoliaceae) and Pinus densiflora (Pinaceae), and deciduous trees such as Lyonia ovalifolia (Ericaceae) and Prunus grayana (Rosaceae) [12] . In the forest, 2-cm segments of terminal roots were randomly sampled from 3 cm below the soil surface at 1-m horizontal intervals within a 59 × 15 m 2 plot from 1 July to 7 July 2010. As the sampling was indiscriminate in terms of root morphology and mycorrhizal type, the samples included roots potentially colonized not only by mycorrhizal fungi but also by diverse root-endophytic and parasitic fungi. Sequences of plant chloroplast rbcL and fungal internal transcribed spacer (ITS) regions were obtained from 834 randomly collected root samples, which represented the root–hyphal associations of 33 plant species and 387 fungal OTUs [12] ( Supplementary Data 1 ). Among the fungal OTUs, 85 OTUs were possibly ectomycorrhizal and 10 were arbuscular mycorrhizal, while the ecological roles of the remaining OTUs could not be inferred due to the lack of reference information in public DNA databases [12] . The overall data set included 184 OTUs of Ascomycota, 128 Basidiomycota, 10 Glomeromycota and one Chytridiomycota. The remaining OTUs were unidentified even at phylum level due to the lack of sequence information in public DNA sequence databases [12] . Network architecture Rows and columns within the interaction matrix (Data S5 in the data source study [12] ) represented plant species and fungal OTUs, respectively. Each cell in the matrix included the number of root samples in which the focal plant–fungus association was observed [12] . The architecture of the plant–fungus network was visualized based on the Kamada-Kawai node-layout algorithm using the program Pajek ( http://vlado.fmf.uni-lj.si/pub/networks/pajek/ ). We evaluated the structure of the plant–fungus network using the H 2 ′ metric of specialization [11] , interaction evenness [40] (with the ‘prod’ option [41] ) and nestedness [42] , [43] using the ‘bipartite’ v.2.04 package [41] of R v.3.0.2. Among various indices of nestedness, NODF nestedness [42] , [43] , [44] is commonly used in ecological network studies. The NODF index was originally proposed to evaluate the nestedness of ‘binary’ network matrices, in which the absence/presence of interactions between pairs of species are represented in a binary (0/1) data format [43] . However, the NODF method can be applied to ‘quantitative’ network matrices, in which elements for respective pairs of species represent the relative frequencies of interspecific interactions [42] . The statistical results based on the two nestedness metrics were consistent with each other (weighted NODF, Fig. 3 ; binary NODF, Supplementary Fig. 2 ). The significance level of each network index was examined by randomization analyses. As most network parameters are associated with connectance [20] , [45] , randomization tests were conducted with the ‘vaznull’ algorithm [46] that kept the species richness, marginal totals (column and row sums in an interaction matrix) and connectance of randomized matrices as observed in original matrices (Model 1; 1,000 permutations; Fig. 3 ; Supplementary Figs 2 and 6 ). The use of an algorithm that could change the connectance of randomized matrices (‘r2dtable’ algorithm [41] ) did not qualitatively alter the results (Model 2 in Supplementary Table 1 ). We further confirmed the statistical results by conducting another type of randomization. In the original community data matrix showing the presence/absence of each fungal OTU for each root sample (Data S4 in the data source study [12] ), we randomized the label of plant species among root samples and then converted the randomized sample-level matrices into interaction (that is, plant species x fungal OTU) matrices. The results of the third null model analysis (Model 3) were consistent with those of Models 1 and 2 ( Supplementary Table 1 ). We also determined whether the plant–fungus network was statistically compartmentalized by conducting a modularity analysis based on simulated annealing optimization of modularity metrics [47] using the program MODULAR [48] with 1,000 randomizations based on each of the three null models. For the original data matrix, we performed 50 simulated annealing runs with different random seed numbers, and a modularity estimate was obtained as the mean over the 50 runs. Two types of modularity metrics, of which one was developed for unipartite data matrices (Newman and Girvan’s metric [49] ; Fig. 3 ) and the other for bipartite data matrices (Barber’s metric [50] ; Supplementary Fig. 2 ), returned qualitatively and quantitatively similar results ( Supplementary Table 1 ). To examine the pattern of links in the plant–fungus network in more detail, we analysed whether the composition of hosts and symbionts differentiated within each assemblage [51] . As the network was highly asymmetric (11.7 fungal OTUs/plant sp. ), we predicted that a more distinct sign of intra-trophic-level competition for partners (that is, partner differentiation) would be observed for fungi than for plants. Differentiation of plant species within the fungal community and that of fungal symbiont taxa within the plant community was separately tested based on the ‘checkerboard’ score [51] . For each network or partial network (see below) data set, a randomization test of checkerboard score was performed with each of the three null model algorithms mentioned above (1,000 permutations; Supplementary Fig. 2 ). Comparative analysis of network architecture To compare the connectance and modularity of the below-ground plant–fungus network with those of previously investigated ecological networks, we compiled the data sets of various forms of ecological interaction ( Supplementary Table 2 ). The data set included 51 plant–pollinator, 25 plant–seed disperser, 4 myrmecophyte plant–ant, 3 anemone–anemonefish, 4 plant–herbivore, 7 host–parasite and 27 prey–predator (food web) networks, whose interaction matrices were available from a previous meta-analytical study [52] and a database of ecological interaction matrices [53] . We also collected network matrices from two mycological studies, each of which investigated the composition of arbuscular mycorrhizal fungal symbionts on more than 10 plant species in a forest [14] , [15] . In one of the arbuscular mycorrhizal studies, a quantitative sampling method allowed the estimation of plant–fungus interaction frequency within a community [54] ( Supplementary Table 2 ). Species richness, connectance and modularity were then calculated for all the 123 networks and subsequently compared with those of the plant–fungus network. In addition, the H 2 ′ metric of interaction specialization and weighted NODF nestedness were calculated for the 47 networks for which quantitative data matrices (that is, network matrices with interaction frequency information) were available ( Supplementary Table 2 ). As the estimates of network indices could be influenced by species richness [2] , [20] , we plotted each of the network indices against the axis of species richness ( Fig. 2 ). We further evaluated the architectural characteristics of the plant–fungus network with a multivariate analysis. In a principal component analysis with a correlation matrix of connectance, H 2 ′ , modularity (Barber’s metric for bipartite data sets [50] ) and weighted NODF nestedness, the plant–fungus and other types of ecological networks were plotted on the principal component surfaces. As sampling intensity of interactions (that is, the total number of observed interaction events) can affect the estimates of network architectural indices [55] , we performed an additional comparative analysis, taking into account the total number of observed interactions in each study. Across the 47 networks with interaction frequency information, connectance, H 2 ′ , modularity (Barber’s metric) and weighted NODF nestedness were regressed on the total number of observed interaction events. In addition, we conducted a principal component analysis with a correlation matrix of the total number of interactions, connectance, H 2 ′ , modularity and nestedness ( Supplementary Fig. 4 ). Functional and phylogenetic partial networks The network structure of functionally or phylogenetically defined partial networks was examined and compared with that of the entire below-ground plant–fungus network. We examined the structure of each functional or phylogenetic ‘partial network’, by categorizing them as follows: ‘mycorrhizal partial network’ (that is, ectomycorrhizal+arbuscular mycorrhizal fungi), ‘ectomycorrhizal partial network’ (ectomycorrhizal fungi), ‘arbuscular partial network’ (arbuscular mycorrhizal fungi), ‘ascomycete partial network’ (Ascomycota fungi) and ‘basidiomycete partial network’ (Basidiomycota fungi). All the network indices applied in the analysis of the entire network architecture were used. Each partial network was composed of fungal OTUs representing a functional or phylogenetic partial group and the plant species they associated with. Cutoff DNA sequence similarities and network architecture The robustness of the network index analyses to the cutoff ITS sequence similarities defining fungal OTUs was examined by additional randomization analyses. In the data set mentioned above, fungal OTUs were defined with a cutoff ITS sequence similarity of 95%, given the intra-specific variability of fungal ITS sequences [56] and the relatively high error rate of 454 next-generation sequencing [12] . Using the source next-generation sequencing data set [12] (DDBJ Sequence Read Archive: DRA000935), we reconstructed two additional data matrices, in each of which fungal OTUs were redefined with a cutoff ITS sequence similarity of 93 or 97% ( Supplementary Data 1 ). The 93 and 97% data matrices included 341 and 454 fungal OTUs, respectively ( Supplementary Data 1 ). The randomization tests of the above-mentioned network indices were conducted for each of the two additional data matrices with the vaznull model ( Supplementary Figs 5 and 6 ). For H 2 ′ interaction specialization, modularity (Newman and Girvan’s metric) and weighted NODF nestedness, the randomization analyses were also applied, respectively, to the data sets defined with cutoff similarities of 91, 89, 87, 85, 83 and 81%. Rarefaction analysis To examine the potential influence of reduced sample size on network index estimates, we performed a sensitivity analysis based on rarefaction. Of the 834 root samples analysed in our study, a fixed percentage of samples were randomly sub-sampled in each rarefaction trial. At each percentage from 10 to 90% at 10% intervals, 100 rarefaction trials were performed. The 95% confidence intervals of connectance, H 2 ′, modularity (Barber’s metric) and weighted NODF nestedness were then calculated based on Student’s t -distribution (df=99) at each rarefaction percentage ( Supplementary Fig. 7 ). In addition, the statistical significance of H 2 ′, modularity and nestedness was examined based on randomization tests with Model 1 (100 permutations) for each rarefaction trial. As this analysis was computationally intensive, it was applied to 20 of the 100 rarefaction trials at each rarefaction percentage ( Supplementary Table 5 ). How to cite this article: Toju, H. et al. Assembly of complex plant–fungus networks. Nat. Commun. 5:5273 doi: 10.1038/ncomms6273 (2014).